Tandem synthesis of alternating polyesters from renewable resources The vast majority of commodity materials are obtained from petrochemical feedstocks. These resources will plausibly be depleted within the next 100 years, and the peak in global oil production is estimated to occur within the next few decades. In this regard, biomass represents an abundant carbon-neutral renewable resource for the production of polymers. Here we report a new strategy, based on tandem catalysis, to obtain renewable materials. Commercially available complexes are found to be efficient catalysts for alternating polyesters from the cyclization of dicarboxylic acids followed by alternating copolymerization of the resulting anhydrides with epoxides. This operationally simple method is an attractive strategy for the production of new biodegradable polyesters. The vast majority of commodity materials are obtained from fossil fuels [1] . However, these resources are limited and many studies predict that all fossil resources will be depleted within a few centuries [2] , [3] , [4] , [5] . In this regard, biomass represents an abundant carbon-neutral renewable resource for the production of biomaterials [6] , [7] , [8] , [9] , [10] , [11] , [12] . Many of these renewable resource polymers can also be rendered biodegradable under the appropriate conditions [1] , [13] , [14] . However, except for polylactide, their high cost hampers their widespread use as bulk polymeric materials, relative to conventional petroleum-based plastics [15] . Recognizing that the raw material cost accounts for up to 50% of the overall production cost of biodegradable polymers [12] , several research groups have directed investigative efforts towards the synthesis of new renewable monomers and the catalytic conversion of these monomers into their corresponding polymers, such as polyesters. Generally, aliphatic polyesters are obtained by either polycondensation or ring-opening polymerization of cyclic esters ( Fig. 1 ) [16] . The latter route restricts the polymer architectures to those of the cyclic esters that are available [17] . Although the nearly unlimited choice of diols and diacids gives access to a much larger range of polymer properties, their direct use in polycondensation reactions is energy intensive and requires drastic conditions to drive the reaction towards high conversion and very accurate comonomer stoichiometries to obtain high-molecular-weight products. In this overall context, organic acids have been suggested as important renewable building blocks because they are available in a minimum number of steps from biorefinery carbohydrate streams [18] . Among them, dicarboxylic acids have received attention as platform chemicals and their potential as monomer precursors is a major challenge that deserves to be explored, even if their overall production cost still remains to be reduced in order to be competitive with petrochemical-derived chemicals [19] . 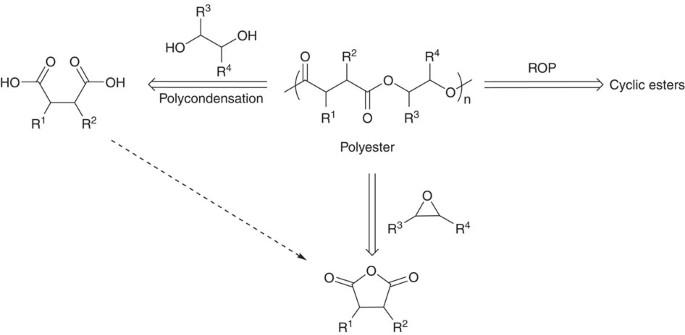Figure 1: Synthetic approaches to aliphatic polyesters. Aliphatic polyesters are obtained by either polycondensation of diols and diacids, ring-opening polymerization of cyclic esters or copolymerization of cyclic anhydrides with epoxides. Figure 1: Synthetic approaches to aliphatic polyesters. Aliphatic polyesters are obtained by either polycondensation of diols and diacids, ring-opening polymerization of cyclic esters or copolymerization of cyclic anhydrides with epoxides. Full size image Tandem catalysis is one of the strategies used by nature for building macromolecules [20] . Living organisms generally synthesize macromolecules by in vivo enzyme-catalyzed chain growth polymerization reactions using activated monomers that have been formed within cells during complex metabolic processes [21] . For instance, aliphatic polyesters, such as polyhydroxyalkanoates, are synthesized from renewable, low-cost feedstocks (for example, sugars or fatty acids) under mild conditions. However, these biological processes rely on highly complex biocatalysts, such as polyhydroxyalkanoate synthases, thus limiting their industrial applications. In the same spirit, we have initiated a research effort to synthesize aliphatic polyesters via an auto-tandem catalytic transformation, where 'activated' monomers (that is, cyclic anhydrides) are synthesized from dicarboxylic acids and subsequently copolymerized with epoxides ( Fig. 1 ). Auto-tandem and assisted tandem catalyses, which make multiple use of a single (pre)catalyst, are more efficient in catalyst utilization than orthogonal catalysis, which requires a different catalyst for each transformation [22] . Although orthogonal tandem catalysis has already been employed for polymer synthesis [23] , [24] , there is no example to date in the literature in which a single metal complex is able to connect two independent catalytic cycles for the production of polymers [25] . Developing a tandem catalytic system is a difficult task, which requires an effective ligand framework for achieving high activity and control during the polymerization reaction and stabilization of the metal centre towards the solvent, substrate, and reaction side products and preventing decomposition of the active species [26] . As pointed out by Jacobsen, salen catalysts (H 2 salen= N , N′ -bis(3,5-di- tert -butylsalicylidene)-1,2-cyclohexanediimine) can be regarded as privileged structures and as useful platforms for the discovery of new reactions [27] . We hypothesized that commercially available metal complexes based on the specific tetradentate salen ligand would have the potential to act as auto-tandem catalysts given their unique robustness and versatility [28] , as well as the documented performance of their chromium counterparts for the synthesis of polycarbonates or polyesters [29] , [30] , [31] , [32] , [33] , [34] . Herein we introduce a practical route to biodegradable polyesters by way of an auto-tandem reaction using simple commercial catalysts. This process provides direct access to anhydrides and polymers in high yields. Cyclization step The first objective of our tandem approach is the synthesis of cyclic anhydrides from dicarboxylic acids. This cyclization is a known transformation, which can only be achieved upon dehydration of the starting compound under acidic conditions and at high temperatures. Accordingly there is a need for a process for the synthesis of cyclic anhydrides, which is fast and, which produces cyclic anhydrides in high yield. Recently Bartoli [35] reported efficient protocols for the preparation of esters from the reaction of carboxylic acids with primary, aromatic and secondary alcohols in the presence of dialkyl dicarbonates under weak Lewis acid catalysis. The mechanism involved a double addition of the acid to the dicarbonate, affording a carboxylic anhydride and an alcohol. The final esters arose from the attack of the alcohols on the anhydrides. Inspired by these previous findings, we envisaged that salen-based catalysts might provide the basis for a multifunctional catalytic system that opens direct access to cyclic anhydrides with high selectivity and flexibility starting from dicarboxylic acids ( Figs 2 , 3 ). 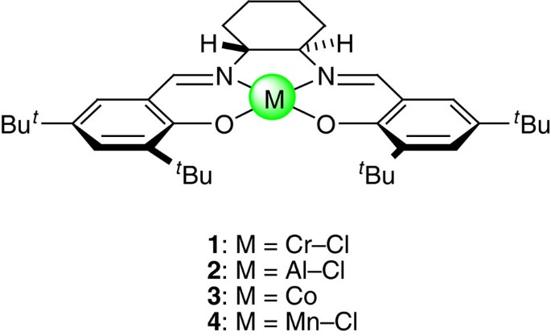Figure 2: Metal-based complexes used. Commercially available metal complexes based on the tetradentate salen ligand are useful platforms for the synthesis of aliphatic polyesters. Figure 2: Metal-based complexes used. Commercially available metal complexes based on the tetradentate salen ligand are useful platforms for the synthesis of aliphatic polyesters. 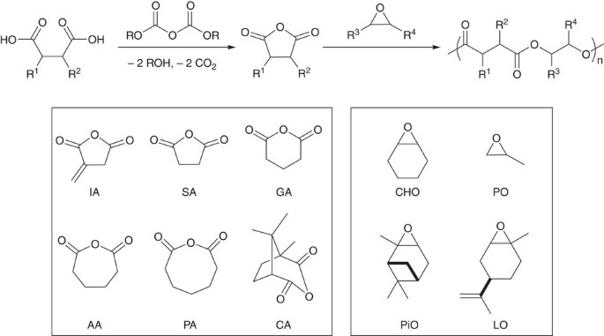Figure 3: Tandem synthesis of polyesters from epoxides and dicarboxylic acids. Salen complexes are efficient catalysts for cyclization of dicarboxylic acids followed by alternating copolymerization of the resulting anhydrides with epoxides. Full size image Figure 3: Tandem synthesis of polyesters from epoxides and dicarboxylic acids. Salen complexes are efficient catalysts for cyclization of dicarboxylic acids followed by alternating copolymerization of the resulting anhydrides with epoxides. Full size image The catalytic performances of the different salen complexes were evaluated in tetrahydrofuran (THF) in the presence of commercially available dialkyl dicarbonates. Representative results are summarized in Table 1 . We first investigated the chromium(III) system 1 . However, the reaction of 100 equiv. of succinic acid with di- tert -butyl dicarbonate (Boc 2 O) in the presence of 1 at 40 °C was unsuccessful. When succinic acid and diethyl dicarbonate (Eoc 2 O) were allowed to react with complex 1 in THF at 40 °C (1 mol%), succinic anhydride (SA) was obtained in 12% yield in 50 h. Gratifyingly, in the presence of dimethyl dicarbonate (Moc 2 O), SA was detected in 100% yield after 10 h. As a control experiment the reaction was performed using a complex in the absence of dicarbonate or using a dicarbonate without a complex, and no reaction product could be isolated after an even longer period of time. We also observed that the addition of cocatalyst [PPN]Cl ([PPN] + =bis(triphenylphosphoranylidene)iminium) increased the catalytic activity (entry 4). These results indicate that the chromate complexes derived from (salen)CrCl and onium salt should be the active species [36] . It has already been demonstrated that this type of Lewis basic cocatalyst reversibly coordinates to the metal centre, increases the electron density on the metal and labilizes the trans ligand to it [37] . Therefore a more electron-rich metal centre is more efficient for this reaction, which is in accordance with Bartoli's observations that the reaction pathway is influenced by the Lewis acidity and that weak Lewis acids are preferable for this reaction [35] . Under the same reaction conditions we were also able to synthesize glutaric (GA), adipic (AA), itaconic (IA), pimelic (PA) and camphoric (CA) anhydrides (entries 5–9). However, for succinic, adipic, glutaric and pimelic acids, we observed that ester formation might occur from attack of alcohol to the anhydride. Thus the reaction had to be stopped before the formation of ester from the corresponding anhydride. For instance, in the presence of complex 1 , pimelic anhydride was detected in 97% yield after 30 min at room temperature, together with the corresponding monoester (3%). Surprisingly in the case of camphoric ( Supplementary Figs S1–S4 ) and itaconic anhydrides no ester formation was detected (entries 8–9). Therefore, under these conditions, strict control of the reaction time was not necessary, as no alcoholysis of the anhydride was observed even after a prolonged reaction time. To avoid alcoholysis of the anhydrides complex 2 was tested as a cyclization catalyst under the same reaction conditions and ester formation was also detected after the reaction (entry 10). However, the reaction of 100 equiv. of pimelic acid with Boc 2 O (instead of Moc 2 O) in the presence of 2 at 50 °C was quantitative and showed no evidence of esterification by 1 H NMR spectroscopy, owing to the much lower nucleophility of tertio -butanol (entry 11). By using the other salen derivatives 3 – 4 , we were also able to completely convert the camphoric acid into the corresponding anhydride (entries 13–14). Thus, the cyclization of dicarboxylic acids with commercially available dicarbonates can be carried out under mild conditions, is rapid in processing and suitable for the preparation of relevant monomers. Only volatile by-products are removed between the anhydride formation step and the copolymerization step so that the resulting monomers are ready for polymerization without purification; thus, a wide range of aliphatic polyesters can be synthesized for different applications. Table 1 Cyclization of dicarboxylic acids. Full size table Polymerization step With an efficient and quantitative synthesis of cyclic anhydrides in hand, we investigated the alternating copolymerization of a series of anhydrides and epoxides using complexes 1 – 4 . The results are summarized in Table 2 . The copolymerizations were performed either in bulk (entries 1–8, 16–18) or in a toluene solution (entries 9–15). Neat conditions were optimal for reactions performed without toluene. The resultant polymers reveal narrow molecular-weight distributions and experimental number-average molecular masses ( M n ) close to the theoretical ones. However, in some cases, experimental M n values do not correspond well with calculated M n values. This mismatch possibly arises from the presence of trace amounts of hydrolyzed anhydride, as already reported by Coates and co-workers [34] . To evaluate the feasibility of the overall process, we conducted preliminary experiments with the chromium-based catalyst 1 , camphoric acid as a model substrate and 1500 equiv. of propylene oxide (PO) as an inexpensive comonomer [38] , [39] , [40] . The Cr(salen) complex was not an effective initiator without co-catalyst (entry 1). However, in the presence of 1 equiv. of PPNCl, this complex was found to be an active initiator for the copolymerization of PO and CA to afford poly(propylene camphorate) ( Supplementary Figs S5–S8 ) with high M n and narrow molecular weight distribution (entry 2). In agreement with previous observations [41] , [42] , [43] , we considered that copolymerization takes place via a mechanism similar to the one reported for the alternating copolymerization of epoxide with CO 2 . The formation of the anionic six coordinate species of the form trans -(salen)CrX 2 − occurs upon treating (salen)CrCl with PPNCl. The next step in the process involves binding and subsequent ring opening of the cyclic ether monomer. The role of the Lewis base cocatalyst is to labilize the metal-nucleophile bond of either the initiator or growing polymer chain towards heterolytic bond cleavage [36] . We then explored other anhydrides as comonomers and found that SA copolymerizes with PO (entry 3) ( Supplementary Figs S9–S12 ). In addition glutaric anhydride and pimelic anhydride react with PO to give polyesters with a moderate M n (entries 4–5) ( Supplementary Figs S13–S20 ). Although the Mn(salen) complex 4 displayed poor reactivity (entry 8) [44] , the screen did reveal the rather surprising result that the cobalt and aluminium analogues catalyzed the alternating copolymerization with similarly good reactivity (entries 6–7). Other epoxides, including cyclohexene oxide (CHO), limonene oxide (LO) and pinene oxide (PiO) are also viable monomers for copolymerization with CA ( Supplementary Figs S21–S28 ); in that case, higher temperature and a longer reaction time are required (entries 9–18). In the presence of 2 equiv. of PPNCl in toluene, the Al(III) complex 2 and the Co(II) complex 3 were more effective catalysts than the chromium analogue 1 for the copolymerization of CHO and CA. This prompted us to investigate the catalytic behaviour of 2 and 3 for the copolymerization of CA and LO. Less reactive alicyclic epoxides, such as α-PiO or LO, are particularly interesting substrates based on biorenewable resources. In particular the pendant functionality of LO provides an opportunity to tune the properties of the resulting polyester through postpolymerization modification of the pendant vinyl groups. In that case the aluminium derivative 2 was found to be much more active than the cobalt catalyst 3 , as it converted 85% monomers in 28 h versus 29% in 28 h for 3 (entries 12, 13). Optimization of the molar ratio between aluminium complex and [PPN]Cl revealed that the highest activity was achieved when using more than 2 equiv. of [PPN]Cl (entries 13, 15–18). Other counteranions for [PPN] + , such as azide, acetate and perfluorobenzoate, can be also employed without a significant influence on catalytic activity. This is in accordance with previous studies that demonstrated that the formation of the six coordinate anion trans -(salen)MX 2 − occurs more easily with at least 2 equiv. of PPNCl. [36] Notably, the combination based on aluminium complex 2 and 5 equiv. of PPNCl in bulk LO was also very reactive (entry 16). Finally it was interesting to observe that aluminium complex 2 is also active for the copolymerization of glutaric anhydride and PiO; neat conditions were optimal for this reaction. To the best of our knowledge, this is the first copolymer synthesized from PiO (entry 17). Table 2 Tandem synthesis of aliphatic polyesters. Full size table As control experiments, we performed polymerization reactions using a clean combination of isolated anhydrides with epoxides in the presence of the precatalyst ( Table 3 ). Interestingly, we observed that direct synthesis gives polymers with similar molecular weights and approximate rates as the tandem system ( Table 2 , entries 3–4). These results suggest that the active species formed during the copolymerization process might be the same species in the overall tandem process (that is, trans -(salen)MX 2 − ). Table 3 Alternating copolymerization of epoxides and isolated cyclic anhydrides. Full size table We have introduced a new class of tandem catalysts for the synthesis of biodegradable polyesters. Insight into the mechanism of individual catalytic cycles, and the resulting ability to control turnover frequencies need to be further developed in this context. The discovery of efficient and selective tandem catalysts for the synthesis of renewable polymers is a crucial requirement for the sustained growth of the chemical industry. Increasingly important will also be the stereoselective catalysts that provide key enantiomerically pure monomers for the design and preparation of novel stereoregular macromolecules as promising advanced commodity materials in a sustainable development context. These results suggest a number of new avenues for next generation renewable polymers. Materials (+)-Limonene oxide (mixture of cis and trans ), propylene oxide, CHO and α-PiO (all purchased from Aldrich) were stirred over calcium hydride, put through three freeze-pump-thaw cycles, then vacuum transferred under argon (twice) and stored in a glovebox. (1 R ,3 S )-(+)-Camphoric acid, glutaric acid (purchased from Aldrich), pimelic acid and succinic acid (purchased from Janssen Chimica) were recrystallized three times with THF/pentane or methylene chloride/diethyl ether, dried overnight under vacuum and then stored in the glovebox. Dimethyl dicarbonate, diethyl dicarbonate and di- tertio -butyl dicarbonate (purchased from Aldrich) are degassed by freeze-thaw-vacuum cycles and stored in the freezer of the glovebox. (1 R ,2 R )-(−)-[1,2,-Cyclohexanediamino- N , N ′-bis(3,5-di- tertio -butylsalicylidene)]chromium(III) chloride, aluminium(III) chloride and manganese (III) chloride were purchased from Strem Chemicals and used as received in the glovebox. (1 R ,2 R )-(−)-[1,2,-Cyclohexanediamino- N , N ′-bis(3,5-di- tertio -butylsalicylidene)]cobalt(II) was purchased from Aldrich, and used as received in the glovebox. Bis(triphenylphosphoranylidene)ammonium chloride (purchased from Fluka) was recrystallized twice with acetone/pentane or methylene chloride/pentane, dried overnight under vacuum and then stored in the freezer of the glovebox. Tandem procedure A Schlenk flask was charged with a solution of the catalyst (10 μmol), PPNCl (6 mg, 10 μmol), dicarboxylic acid (1 mmol) and dimethyl dicarbonate (1 mmol, 110 μl, 134 mg) in 1 ml of THF. The solution was stirred at 40 °C. After the allocated reaction time, the reaction was checked by 1 H NMR spectroscopy, which indicated complete and selective conversion of the starting dicarboxylic acid. When the conversion is complete, volatiles are removed under vacuum overnight. The complex was directly engaged in polymerization after the addition of a solution of epoxide in the appropriate ratio in toluene. The reaction was stirred at the desired temperature for the desired reaction time. After a small sample of the crude material was removed for characterization, the reaction was quenched with acidic methanol (0.5 ml), and the polymer was precipitated with excess of pentane. The polymer was then dried in vacuo to constant weight. Measurements All manipulations requiring dry atmosphere were performed under a purified argon atmosphere using standard Schlenk techniques or in a glovebox. Solvents (toluene, pentane, THF) were freshly distilled from Na/K alloy under nitrogen and degassed thoroughly by freeze-thaw-vacuum cycles before use. Deuterated solvents (benzene- d 6 , toluene- d 8 , THF- d 8 /99.5% D, Eurisotop) were freshly distilled from sodium/potassium amalgam under argon and degassed before use. NMR spectra were recorded on Bruker Avance-300, Avance-400 and Avance-600 spectrometers. 1 H and 13 C chemical shifts are reported in p.p.m. versus SiMe 4 and were determined by reference to the residual solvent peaks. Assignment of signals was made from multinuclear 1D ( 1 H, 13 C{ 1 H}) and 2D (correlation spectroscopy, heteronuclear multiple quantum coherence, heteronuclear multiple bond correlation) NMR experiments. Gel permeation chromatography analyses were carried out using a Waters instrument GPCV 2000, equipped with an ultraviolet and a viscometry detectors. The columns used are Styragel columns (two HT6E and one HT2) filled with 10 μm styrene-divinyl benzene gel balls. The number average molecular masses ( M n ) and polydispersity index ( M w / M n ) of the resultant polymers were calculated with reference to a polystyrene calibration. IR analyses were carried out using a FT/IR-4100 Jasco instrument, with a ATR PRO450-S, a TGR detector, 2 mm per sec scanning speed and a resolution of 16 cm −1 . How to cite this article: Robert, C. et al . Tandem synthesis of alternating polyesters from renewable resources. Nat. Commun. 2:586 doi: 10.1038/ncomms1596 (2011).